Large-scale solution synthesis of narrow graphene nanoribbons According to theoretical studies, narrow graphene nanoribbons with atomically precise armchair edges and widths of <2 nm have a bandgap comparable to that in silicon (1.1 eV), which makes them potentially promising for logic applications. Different top–down fabrication approaches typically yield ribbons with width >10 nm and have limited control over their edge structure. Here we demonstrate a novel bottom–up approach that yields gram quantities of high-aspect-ratio graphene nanoribbons, which are only ~1 nm wide and have atomically smooth armchair edges. These ribbons are shown to have a large electronic bandgap of ~1.3 eV, which is significantly higher than any value reported so far in experimental studies of graphene nanoribbons prepared by top–down approaches. These synthetic ribbons could have lengths of >100 nm and self-assemble in highly ordered few-micrometer-long ‘nanobelts’ that can be visualized by conventional microscopy techniques, and potentially used for the fabrication of electronic devices. Because of its extraordinary electronic, mechanical, thermal and optical properties, graphene is often considered as a complement, and in some cases even a replacement for silicon in future electronics [1] , [2] , [3] . However, the absence of an energy bandgap in graphene prevents its use in logic applications [2] , [3] . Theoretical studies predict a bandgap comparable to that in silicon (1.1 eV) in narrow graphene nanoribbons (GNRs) that have atomically precise armchair edges and widths <2 nm (refs 4 , 5 ). Different top–down fabrication approaches, such as nanofabrication [6] , [7] , sonochemical method [8] , nanowire lithography [9] , [10] , nanoscale cutting of graphene using nickel nanoparticles [11] , [12] or a diamond knife [13] and unzipping of carbon nanotubes [14] , [15] , [16] , [17] , [18] , [19] , typically yield ribbons with width >10 nm and have limited control over their edge structure. Although several groups demonstrated that such GNRs could exhibit an insulating state in electrical measurements, it was later argued that the observed transport bandgaps of up to ~200–400 meV (refs 7 , 8 , 9 ) are likely to be caused by strong localization effects due to edge disorder, rather than a true gap between valence and conduction bands [20] , [21] , [22] . Thus, it is important to develop techniques to produce large quantities of GNRs that are only 1–2 nm wide and have atomically precise armchair edges. Large quantities of GNRs could be prepared by chemical vapour deposition, but the widths of such ribbons (20–300 nm) are too large to open a substantial electronic bandgap [23] . Narrow sulfur-terminated GNRs have been synthesized by decomposition of fullerenes or other molecular precursors inside carbon nanotubes [24] , [25] , but the large-scale production of such ribbons, their separation from the host tubes and subsequent use for electronic devices are very challenging. Recently, Cai et al. [26] have demonstrated that bottom–up chemical approaches have a great potential for the synthesis of narrow GNRs. Ribbons that are only a few benzene rings wide and have atomically smooth armchair edges were synthesized on a surface of either Au (111) or Ag (111) single crystal by coupling molecular precursors into linear polyphenylenes followed by cyclodehydrogenation. This work demonstrates that bottom–up techniques could yield narrow atomically engineered GNRs that are currently unachievable by any top–down approach, stimulating their detailed characterization [27] , [28] , [29] , [30] , [31] , [32] , [33] , [34] , as well as further research and development of new synthetic methods for GNRs. Of particular interest are novel solution-based approaches, which, in contrast to surface-limited coupling techniques, could yield bulk quantities of GNRs for large-scale applications [35] , [36] , [37] , [38] , [39] , [40] . Also, GNRs prepared on a conductive Au (111) or Ag (111) single crystal cannot be directly used for device fabrication and electrical testing, and thus should be somehow transferred to a dielectric substrate, while GNRs synthesized in solution could be conveniently deposited on any substrate of choice, such as Si/SiO 2 . Here we report a solution-based synthetic approach for large quantities of GNRs that are ~1 nm wide, could have length >100 nm and self-assemble in highly ordered micrometer-long superstructures. These GNRs and especially their assemblies are long enough to bridge nanogaps fabricated by the standard electron-beam lithography (EBL) [41] , [42] . Synthesis of GNRs A particular GNR that we attempted to fabricate in this work is shown in Fig. 1a ; it has a width of only ~1 nm and uniform armchair edges. According to the density functional theory calculations ( Fig. 1b ), this ribbon has an electronic bandgap of ~1.6 eV (ref. 26 ); an even larger value would be obtained using an alternative computational approach [27] , [43] . This value is larger than that in silicon (1.1 eV), suggesting that such GNRs could possibly be utilized for the fabrication of field-effect transistors with high on-off ratios. Furthermore, a recent theoretical study suggests that these ribbons ( Fig. 1a ) are very promising materials for optoelectronic applications [44] that will require large quantities of such GNRs. 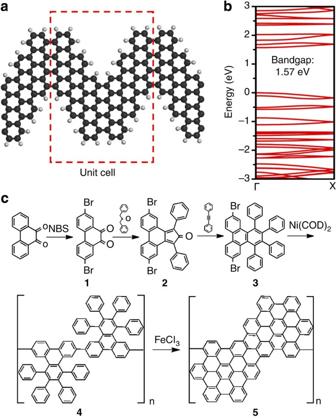Figure 1: Synthesis of GNRs with a large electronic bandgap. (a) Schematic of the GNRs synthesized in this study and (b) the corresponding calculated band structure. (c) Reaction scheme used in this work, see text for details. Figure 1: Synthesis of GNRs with a large electronic bandgap. ( a ) Schematic of the GNRs synthesized in this study and ( b ) the corresponding calculated band structure. ( c ) Reaction scheme used in this work, see text for details. Full size image The reaction scheme used in this work to synthesize these GNRs is shown in Fig. 1c . Briefly, it is based on a polymerization of pre-synthesized molecular precursors by a Ni 0 -mediated Yamamoto coupling [45] followed by a cyclodehydrogenation via a Scholl reaction using iron (III) chloride [46] to form GNRs. This synthetic approach is described in detail in the Methods section. We demonstrate that the procedure is scalable, and over 1 g of ribbons could be synthesized in a single synthesis; see the Supplementary Note 1 . We believe that this approach is very general, and by using other molecular precursors instead of 3 it would be possible to synthesize other GNRs with different widths and geometries [26] . Characterization of GNRs and intermediate products Molecules 1 – 3 were characterized by mass spectrometry (MS) and/or 1 H/ 13 C nuclear magnetic resonance (NMR); see the Methods section and Supplementary Figs 1–6 . Here we discuss the last two steps in the reaction scheme, which are the transformations of molecule 3 to polymer 4 to GNR 5 . First of all, these products have different colours, as shown in the top inset in Fig. 2a . Furthermore, this figure clearly shows that macroscopic quantities of all products, including GNRs, are attainable by the described synthetic approach. All three materials exhibit very different photoluminescence properties. The bottom inset in Fig. 2a shows three vials with products 3 , 4 and 5 dispersed in dichloromethane (DCM) at the same concentration of 0.167 mg ml −1 , which were irradiated with a 365 nm ultraviolet (UV) lamp (note that polymer 4 and GNR 5 do not dissolve in DCM; they could be dispersed by sonication for the measurements but then quickly precipitate). While molecule 3 exhibits only a barely noticeable blue emission, polymer 4 shows a very bright cyan emission and GNRs 5 exhibit no visible emission; photoluminescence spectra of all three products recorded with a 405 nm excitation light ( Fig. 2a ) agree well with these observations. Thus, optical and photoluminescence data confirm a significant structural difference between products 3 , 4 and 5 . 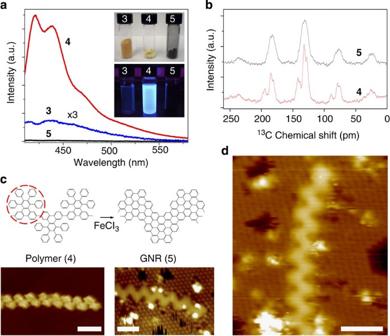Figure 2: Comparison of GNRs and intermediate reaction products. (a) Photoluminescence spectra of the molecule3, polymer4and GNRs5; spectrum3is magnified by factor 3 for clarity. The top inset shows 5 ml vials with all three products; the bottom inset shows 5 ml vials with 0.167 mg ml−1dispersions of the same products in DCM, irradiated from the back by a 365 nm ultraviolet lamp; numbers on the vials correspond to the numbers inFig. 1c. (b)13C NMR spectra for the polymer4and GNRs5. (c) Atomic structures and corresponding STM images of a polymer4and a GNR5deposited on an Au (111) single crystal. Scale bars, 3 nm. (d) STM image of another GNR5on Au (111). Scale bar, 3 nm. Figure 2: Comparison of GNRs and intermediate reaction products. ( a ) Photoluminescence spectra of the molecule 3 , polymer 4 and GNRs 5 ; spectrum 3 is magnified by factor 3 for clarity. The top inset shows 5 ml vials with all three products; the bottom inset shows 5 ml vials with 0.167 mg ml −1 dispersions of the same products in DCM, irradiated from the back by a 365 nm ultraviolet lamp; numbers on the vials correspond to the numbers in Fig. 1c . ( b ) 13 C NMR spectra for the polymer 4 and GNRs 5 . ( c ) Atomic structures and corresponding STM images of a polymer 4 and a GNR 5 deposited on an Au (111) single crystal. Scale bars, 3 nm. ( d ) STM image of another GNR 5 on Au (111). Scale bar, 3 nm. Full size image Figure 2b illustrates structural transformations that occur by cyclodehydrogenation of polymer 4 to form GNRs 5 , as observed by 13 C NMR. In polymer 4 the solid state 13 C spectrum shows two groups of resonances: one at 140 p.p.m. and one at 130 p.p.m. All other resonances within the spectrum are spinning sidebands of these peaks at multiples of 8,000 Hz (rotor spinning rate) from these two groups of resonances. The broad peak at 140 p.p.m is the ipso carbons in aromatic ring- sp 2 hybridized carbons attached to other carbons. The broad peak at 130 p.p.m is from sp 2 hybridized carbons attached to protons. Polymer 4 loses some of these protons in the Scholl reaction to form 5 . Most carbons within 5 are bonded to other carbons, which broadens the signal to the average resonance at 130 p.p.m. Again all the other peaks in the 13 C spectrum for 5 are spinning sidebands at the rotor resonance period (8,000 Hz). Microscopic characterization of GNRs We also confirmed the successful transformation of the polymer 4 to GNR 5 by scanning tunnelling microscopy (STM), see Fig. 2c . Bottom left panel in Fig. 2c shows an STM image of a polymer 4 deposited on an Au (111) single crystal. In accordance with the atomic structure of the polymer, it demonstrates regions of high electron density that correspond to molecular fragments shown by the red circle in Fig. 2c . Furthermore, the polymer does not appear to be flat, which is in a good agreement with prior works: it was reported that phenyl groups of a polymer deposited on a gold substrate are tilted with respect to the surface and thus result in bright features in STM images [26] . In contrast to polymer 4 , GNRs 5 appear to be perfectly flat on a Au (111) substrate, and the electron density is evenly distributed along the ribbon, which is expected for a fully aromatic system (see Fig. 2d and bottom right panel in Fig. 2c ). The structure of the ribbons observed in these STM images is in perfect agreement with the atomic structure of a GNR 5 . Since these GNRs were deposited on an Au (111) single crystal in air from a toluene solution, it is inevitable that some solvent residues and other surface adsorbates will remain on the gold surface even in the high-vacuum STM chamber. Thus, we attribute occasional white spots in STM images reported in this work to such adsorbates. Also, it should be noted that in order to prepare a sample for the STM analysis the GNRs should be heavily sonicated in an appropriate solvent, such as toluene, to be well dispersed. However, sonication is known to cut GNRs that are even 1–2 orders of magnitude wider than the ones reported in this work [14] . Therefore, Fig. 2d and similar STM images of heavily sonicated ribbons cannot be used to assess the lengths of these GNRs in a solution. If the ribbons are not heavily sonicated but dispersed in toluene in milder conditions, deposited on a substrate and imaged by atomic force microscopy (AFM) upon drying, a very different morphology of GNRs is observed. 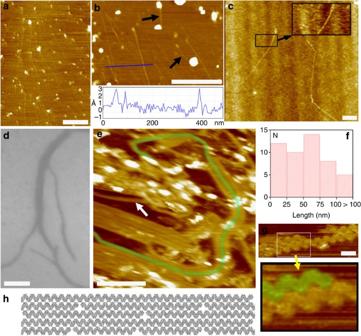Figure 3: Microscopy characterization of GNRs. (a,b) AFM images of GNRs deposited on mica. Bottom panel in (b) shows the height profile along the blue line. Scale bars, 500 nm. (c) AFM image of GNRs deposited on a Si/SiO2substrate. Scale bar, 1 μm. (d) SEM image of GNRs deposited on a Si/SiO2substrate. Scale bar, 200 nm. (e) STM image of GNRs deposited on an Au (111) single crystal and annealed under vacuum at 40 °C for 20 min inside the STM chamber prior to imaging. The GNR highlighted in green is ~80 nm long. Scale bar, 10 nm. (f) Size distribution of the lengths of individual GNR observed in multiple STM images. (g) STM image showing arrangement of GNRs. Scale bar, 3 nm. In the magnified part one GNR is highlighted in green for the sake of clarity. (h) The proposed structure of a GNR nanobelt. Note that this schematic does not represent the actual lengths of individual GNRs. Figure 3a–c shows representative AFM images of GNRs deposited on a freshly cleaved surface of mica and on a Si/SiO 2 substrate; additional images are shown in the Supplementary Fig. 7 . Observed in such images are elongated structures that are thin and remarkably long; many of them have lengths >1 μm. Because of their large size, we could not determine the molecular mass of these structures by MS. These structures could be mistaken for individual GNRs, but we demonstrate below that these structures are actually ‘nanobelts’ of GNRs attached in a side-by-side fashion. The structure of these nanobelts was determined by a combination of microscopy techniques such as AFM, scanning electron microscopy (SEM) and STM. Figure 3: Microscopy characterization of GNRs. ( a , b ) AFM images of GNRs deposited on mica. Bottom panel in ( b ) shows the height profile along the blue line. Scale bars, 500 nm. ( c ) AFM image of GNRs deposited on a Si/SiO 2 substrate. Scale bar, 1 μm. ( d ) SEM image of GNRs deposited on a Si/SiO 2 substrate. Scale bar, 200 nm. ( e ) STM image of GNRs deposited on an Au (111) single crystal and annealed under vacuum at 40 °C for 20 min inside the STM chamber prior to imaging. The GNR highlighted in green is ~80 nm long. Scale bar, 10 nm. ( f ) Size distribution of the lengths of individual GNR observed in multiple STM images. ( g ) STM image showing arrangement of GNRs. Scale bar, 3 nm. In the magnified part one GNR is highlighted in green for the sake of clarity. ( h ) The proposed structure of a GNR nanobelt. Note that this schematic does not represent the actual lengths of individual GNRs. Full size image Using AFM we can precisely determine the heights of such GNR nanobelts. The bottom panel in Fig. 3b shows a representative height profile across two of these nanobelts, one of which is folded. Both nanobelts have a height of ~3 Å, which is very close to the interlayer spacing in graphite (3.35 Å) [47] . We have measured height profiles in different AFM images for >80 such nanobelts (several additional height profiles are shown in the Supplementary Fig. 7 ), and in all cases we have observed heights <5 Å. This means that these nanobelts are not stacks of GNRs, because their thickness corresponds to the thickness of a single graphene ribbon. The inset in Fig. 3c shows two GNR nanobelts that have a similar height of ~4 Å but visibly different widths. While AFM cannot be used for a precise measurement of widths of these GNR nanobelts because of the tip curvature effect, such information could be obtained by SEM. A representative SEM image ( Fig. 3d ) confirms that GNR nanobelts have different widths that range from only a few nm to ~60 nm. The narrowest GNR nanobelt visible in Fig. 3d is ~10 nm wide, which corresponds to 5–6 GNRs arranged side by side. To gain further insights into the structure of these GNR nanobelts, we used a toluene dispersion of GNRs that was only mildly agitated and refluxed to prepare a sample for the STM analysis. The sample was annealed at 40 °C for 20 min in vacuum inside the STM chamber prior to imaging to remove some of the residual solvent molecules and atmospheric adsorbates; a typical STM image is shown in Fig. 3e . In this series of experiments we could not resolve fine structural features of GNRs like in Fig. 2d , but numerous sub-2-nm strands that we attribute to individual ribbons are clearly visible; one of these ribbons is indicated by the white arrow. Such images confirm that GNRs indeed tend to form side-by-side assemblies that comprise 3–7 individual ribbons. Using Fig. 3 and similar STM images it was also possible to size individual GNRs that were not heavily sonicated in a solution. We found ca . 50 GNRs for which we could observe both ends and measured their lengths; the resulting size distribution is shown in Fig. 3f . Some GNRs were >50 nm long (for example, the GNR highlighted in green in Fig. 3e is ~80 nm long) and several were >100 nm long (see one example in the Supplementary Fig. 8 ); such GNRs are long enough to bridge electrodes fabricated by standard EBL technique [41] (nanogaps as small as 10 nm with high aspect ratios could be fabricated by some modified EBL-based techniques [42] ). Higher magnification STM images reveal the actual arrangement of individual GNRs in nanobelts. Figure 3g shows that when GNRs are arranged in a side-by-side fashion, the protrusions of one ribbon perfectly fit into the grooves of another one. Thus, based on the results of AFM, SEM and STM we conclude the observed GNR nanobelts consist of several ribbons attached side by side as shown in Fig. 3h . At the moment it remains unclear whether these structures exist in solution or form directly on a substrate by capillary forces during the solvent evaporation; it is also unclear whether this side-by-side attachment is the only possible type of GNR assembly, or some of the ribbons in certain conditions also assemble via the π–π stacking or form ‘slanted’ structures [48] ; these questions will be answered in future studies. Figure 3a shows these GNR nanobelts span from the bottom part of the image to its top left corner; similarly aligned nanobelts are observed in panel (b). The GNR nanobelts were possibly straightened and partially aligned in the contact angle between a solution droplet and the surface of a substrate during the solvent drying. Possible alignment of GNR nanobelts could streamline the device fabrication in future studies [49] . Furthermore, since GNR-based electronic devices are typically fabricated on Si/SiO 2 substrates [6] , [7] , [8] , [9] , [10] , [14] , [15] , [18] , [20] , [21] , it is important that these GNR nanobelts, although only a few angstroms thick, could be visualized by AFM not only on atomically flat mica but also on substrates with a rougher surface, such as Si/SiO 2 ( Fig. 3c ). Because of their large size, some of these GNR nanobelts could aggregate or entangle. For example, the black arrows in Fig. 3b shows two nanobelts with entangled ends; the entangled parts of the GNR nanobelts look like white spots in the AFM image. We have occasionally observed similar white spots at the ends and even in the middle of some nanobelts in other AFM images (see the Supplementary Fig. 7 ). Some of these nanobelts are fully entangled and appear as larger white spots in AFM images ( Fig. 3a,b ). However, the majority of nanobelts in these AFM images appear to be straightened and not entangled. Spectroscopic characterization of GNRs We have further characterized GNRs by several spectroscopic techniques. 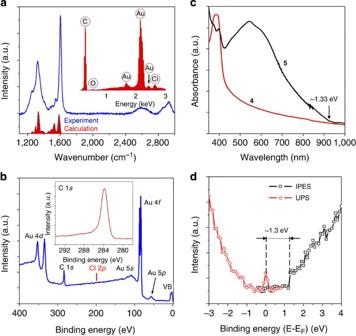Figure 4: Spectroscopic characterization of GNRs. (a) Raman spectrum. The inset shows the EDX spectrum of GNRs deposited on a gold substrate. (b) XPS survey spectrum of GNRs deposited on a gold substrate. The inset shows the XPS C1s spectrum of the same sample. (c) UV–vis-NIR absorption spectra of polymer4(red) and GNRs5(black) suspended in DMF by sonication. (d) UPS/IPES spectrum of GNRs on a gold substrate. Figure 4a demonstrates a Raman spectrum, where the most intense lines of ~1,300 and 1,600 cm −1 , typically referred to as D- and G-bands, respectively [50] , show an apparent fine structure. This pattern is characteristic for all-benzene polycyclic aromatic hydrocarbons (PAHs); the relative intensities and positions of the lines depend on the molecular structure of a PAH [51] , [52] . We performed a simulation of the GNR 5 Raman spectrum and found a good agreement between the calculated and experimentally observed peak positions. In accordance with the experiment, the calculated spectrum predicts the fine structure of three separate peaks at the left shoulder of the G band but no additional peaks at the right shoulder. Similarly, the calculated spectrum predicts a small peak at the right shoulder of the D band and larger peaks at the left shoulder; these features are also observed experimentally. Owing to the high sensitivity of the Raman spectroscopy to the disorder in carbon materials, the experimental observation of the fine structure in the Raman spectrum of GNRs could be considered as another evidence to the high structural quality of the synthesized material. Figure 4: Spectroscopic characterization of GNRs. ( a ) Raman spectrum. The inset shows the EDX spectrum of GNRs deposited on a gold substrate. ( b ) XPS survey spectrum of GNRs deposited on a gold substrate. The inset shows the XPS C1s spectrum of the same sample. ( c ) UV–vis-NIR absorption spectra of polymer 4 (red) and GNRs 5 (black) suspended in DMF by sonication. ( d ) UPS/IPES spectrum of GNRs on a gold substrate. Full size image The inset in Fig. 4a shows an EDX spectrum of GNRs deposited on a gold foil. Except for the strong Au peaks that are originated from the substrate, the only foreign peak observed is the low intensity Cl line (atomic ratio C:Cl~300:1), which could be caused by either Cl − ions adsorbed on ribbons after the HCl washing in the last reaction step or DCM that was used for the sample preparation. We also mark the position of the O peak, demonstrating that only a negligible amount of oxygen, which is probably caused by atmospheric adsorbates, could be detected. No other impurity elements from different reagents and catalysts used in the GNR synthesis were detected. Interestingly, chlorine impurities, which were observed by EDX, were not detected by the X-ray photoelectron spectroscopy (XPS) analysis of the same sample ( Fig. 4b ), possibly because the XPS analysis was performed in higher vacuum compared with the EDX, which facilitated the desorption of DCM residues. The XPS survey scan shown in Fig. 4b demonstrates only the peaks associated with the GNRs and the gold substrate. The inset in Fig. 4b shows the XPS C1s spectrum where only a single sharp component at 284.5 eV corresponding to the sp 2 carbons is observed. No other peaks corresponding to the carbon in different oxygen-containing functionalities [53] are observed, further confirming that these GNRs are chemically pure and are not oxidized in air. Figure 4c shows a UV–vis-NIR spectrum of the dispersion of ribbons sonicated in N,N-dimethylformamide (DMF) (along with N-methyl-2-pyrrolidone (NMP) DMF was found to be a very effective dispersion medium for GNRs, see Supplementary Fig. 9 and Supplementary Note 2 ); a spectrum of polymer 4 is shown for comparison. The GNR spectrum exhibits a strong absorption in the UV and visible region, and an absorption edge in NIR. The absorption onset at ~930 nm corresponds to the optically measured bandgap in GNRs of ~1.33 eV (refs 40 , 54 ). This value is significantly higher than other experimental bandgap values reported for GNRs fabricated by top–down approaches [6] , [7] , [8] , [9] , [18] ; it is close to the calculated value of 1.6 eV ( Fig. 1b ) and higher than that in silicon (1.1 eV). To better assess the bandgap in these GNRs, we have performed combined ultraviolet photoemission spectroscopy (UPS) and inverse photoemission spectroscopy (IPES). The measurements were performed on a pressed pellet of GNRs that was 0.75 cm in diameter and ~0.5 mm thick ( Supplementary Fig. 10 ); the pellet was placed on a Au (111) surface that was also used for the spectrometer calibration. The combined UPS/IPES measurements were undertaken to study the molecular orbital placement of both occupied and unoccupied orbitals in GNRs. In both UPS and IPES measurements, the binding energies were referenced with respect to the Fermi edge of gold in intimate contact with the samples studied, so as to correctly establish the chemical potential free of all instrumental errors. The data are shown in terms of E – E F , thus making occupied state energies negative. The UPS/IPES data are shown in Fig. 4d ; qualitatively similar energy spectra were previously measured by the scanning tunnelling spectroscopy for other GNRs synthesized by a surface-assisted approach [27] , [30] . We have observed a bandgap of ~1.3 eV, which is in good agreement with the results of optical spectroscopy. The observed peak in the UPES spectrum (occupied density of states) that appears at the Fermi level could be a result of the fact that these GNRs have large effective mass (as expected) leading to a large density of states at the top of the valence band maximum. Narrow occupied states of heavy effective mass could also emerge from edge states that are a direct result of the restricted dimensionality of the GNR; similar peaks in scanning tunnelling spectroscopy spectra of other GNRs were also interpreted as the edge states [55] , [56] . This occupied state observed in the UPES spectrum at the Fermi level may in fact be more narrow than plotted in Fig. 4d , as there is finite instrumental resolution of >70 meV and the measurements done at the elevated temperature of 300 K, adding a thermal broadening widths to the GNR states observed, in addition to any lifetime broadening and band dispersion broadening effects. In spite of an extremely low density of occupied states in the vicinity of the chemical potential, this material is p-type, that is, the LUMO is well above the chemical potential ( E F ). The 1.3 eV bandgap of GNRs 5 is close to the optical bandgap of 1.12 eV reported for other solution-synthesized GNRs [40] ; as expected, the value found in the present work is slightly larger because the GNRs 5 are narrower than the ribbons synthesized in ref. 40 . However, the 1.3 eV bandgap is substantially lower than the values reported in the studies of individual GNRs synthesized by the surface-assisted approach on gold substrates [27] , [28] , [33] , [34] . For example, a significantly larger bandgap of 3.1±0.4 eV was recently reported for the same GNRs 5 synthesized on Au(788) by the surface-assisted approach [34] ; this value is much higher than the value of ~1.3 eV found in this work for GNRs 5 , and even larger or comparable to the bandgap of the precursor polymer 4 (~2.9 eV) determined from the absorption onset in the optical spectrum ( Fig. 4c ). A possible explanation for these differences is the fact that the characterization of solution-synthesized GNRs (or polymer precursors), such as UV-vis-NIR and UPS/IPES, is performed on bulk samples where GNRs (or precursor polymers) are heavily aggregated, whereas prior measurements were performed on isolated GNRs on a gold substrate [34] . Aggregation effects were previously shown to affect the optical absorption spectra of PAH molecules visibly reducing their apparent bandgaps [57] . Similarly, it is possible that the value of ~1.3 eV represents not an intrinsic bandgap of an individual GNR 5 but a bandgap of a bulk GNR material. On the other hand, the results of the band structure measurements of GNRs on metallic substrates should be affected by the GNR–substrate interactions (for example, gold was shown theoretically [58] and experimentally [59] to cause the hole doping of graphene), which should also be taken into account when interpreting the data or comparing the results of different experiments. Even if the value of 1.3 eV represents the bandgap of a bulk GNR material, knowing this bandgap is very important, because of many potential bulk applications of synthetic GNRs, such as photovoltaics, printed electronics and composite materials. Additional studies of the band structures of different synthetic GNRs in general and GNR aggregation effects in particular are definitely in order. We have demonstrated a novel bottom–up approach that yields gram quantities of high-aspect-ratio GNRs, which are only ~1 nm wide and have atomically smooth armchair edges. The important characteristics of these GNRs are their large bandgap of ~1.3 eV, their large lengths, the ease with which they can be deposited on any substrate and their ability to be visualized by conventional microscopy techniques. Although we have demonstrated the synthesis of only one type of GNRs, we believe that GNRs with other structures could also be synthesized by a similar bottom–up approach. Further device studies will reveal whether these GNRs with large electronic bandgaps could be used in high on-off ratios field-effect transistors, logic gates and photovoltaic devices. Materials All starting materials and solvents were purchased and used as received without any purification. Phenanthrene-9,10-dione (95%), potassium hydroxide (85%), diphenyl ether (99%), nitromethane (98%), iron (III) chloride (anhydrous, 98%), 1,3-diphenylacetone (98+%), DMF and gold foils (99.985%) were purchased from Alfa Aesar. N-bromosuccinimide (NBS, 99%), diphenylacetylene (98%), bis(1,5-cyclooctadiene)nickel(0), cyclooctadiene (COD), 2,2′-bipyridyl, toluene and methanol were purchased from Sigma-Aldrich. Sulphuric acid (98%) was purchased from EMD. Mica, V4 grade was purchased from SPI Supplies. 4-inch heavily p-doped silicon wafers with a 300-nm-thick layer of SiO 2 were purchased from Silicon Quest International. Synthesis of 1 Synthesis of 1 was adapted from the work by Unver et al. [60] ; 7 g (33 mmol) of phenanthrene-9,10-dione was added to 190 ml of 98% sulphuric acid and followed by the addition of 12.86 g (72 mmol) of NBS. The mixture was agitated at room temperature for 8 h. After stirring, the mixture was added to ice water bath and filtered to obtain a deep orange solid with a quantitative yield. 1 H NMR (300 Hz, DMSO-d 6 ): δ =8.24 (2H, d, J =8.60 Hz), 8.70 (2H, d, J =2.38 Hz), 7.95 (2 H, dd, J =2.30, 8.50 Hz); see Supplementary Fig. 1 . Synthesis of 2 The procedure was adapted and modified from the work by Saleh et al. [61] ; 2.67 g (7.3 mmol) of 1 and 1.85 g (8.81 mmol) of 1,3-diphenylacetone were added to 15 ml methanol under stirring. The reaction mixture was heated to reflux and 25.56 ml of 0.3 M KOH (7.67 mmol) in methanol was added dropwise. The reaction mixture was refluxed for 2 h and then filtered. A total of 2.5 g of green solid was obtained at 63.4% yield. 1 H NMR (600 Hz, CD 2 Cl 2 ): δ =7.65 (2H, d, J =8.60 Hz), 7.61 (2H, d, 1.70 Hz), 7.49 (4H, dd, J =7.10, 7.50 Hz), 7.45 ( 2H, dd, J =6.90, 7.70 Hz), 7.41 (2H, dd, J =1.80, 7.58 Hz), 7.36 (2H, d, J =7.14); see Supplementary Fig. 2 . Synthesis of 3 The procedure was modified from the procedure by Saleh et al. [61] ; 4 g (7.4 mmol) of 2 was refluxed in 4 ml of diphenylether for 3 days. The crude monomer was precipitated in hexanes and slow-recrystallized in a minimal amount of THF at −20 °C for 24 h to obtain 2.2 g of a brown-red solid at 43% yield. 1 H NMR (300 Hz, CDCl 3 ): δ =8.20 (2H, d, J =8.7 Hz), 7.68 (2H, d, J =1.9 Hz), 7.49 (2H, dd, J =1.9, 8.8 Hz), 7.19–7.14 (6H, m), 7.07–7.04 (4H, m), 6.93–6.89 (6H, m), 6.72–6.69 (4H, m); see Supplementary Fig. 3 . 13 C NMR (300 Hz, CDCl 3 ): δ =142.08, 141.46, 140.08, 137.80, 133.08, 132.51, 132.05, 130.51, 129.74, 128.51, 126.98, 126.93, 125.70, 124.7, 120.33; see Supplementary Fig. 4 . HREI m / z (%): 690.04 (100) [M + ] (calculated 690.04); see Supplementary Fig. 5 . If the red-brown solid was re-crystallized again in methanol/DCM mixture an off-white powder with a yellowish tint is obtained, as shown in Supplementary Fig. 6 . However, based on the 1 H NMR data, there is no difference between the red-brown material and the off-white material that was further purified by additional crystallization, see Supplementary Fig. 6 . Therefore, we did not perform second re-crystallization of 3 to achieve a higher yield of the final product. We also want to point out that since we intended to develop a method for the large-scale synthesis of GNRs, crystallization and/or re-crystallization was a preferred route to isolate the material over a difficult, small-scale and labour-intensive column chromatography technique. Synthesis of polymer 4 Ni(COD) 2 (380.7 mg, 1.12 mmol), 175.0 mg (1.12 mmol) of 2,2′-bipyridyl and 200 μl (1.12 mmol) of COD were added to 5 ml of degassed DMF. The reaction mixture was heated to 55 °C and kept for 30 min. Monomer 3 (200 mg, 0.29 mmol) in 6 ml of degassed toluene was added to the reaction flask. The reaction was performed at 80 °C for 2 days. The polymer was precipitated in methanol, filtered and washed with methanol, concentrated HCl, water, 0.5M NaOH solution in methanol, water, acetone and hexane to obtain 102 mg of yellow powder at 66% yield. Synthesis of GNRs 5 Polymer 4 (30.4 mg) was added to 100 ml of DCM. FeCl 3 (250 mg) in 3 ml of nitromethane was added to the reaction mixture and nitrogen was bubbled through the mixture for 24 h. The black solid was filtered and washed with concentrated HCl, 0.5M NaOH solution in methanol, methanol and acetone to obtain 27.6 mg of black powder. Preparation of AFM and SEM samples Approximately 0.5 mg of GNR powder was added to a 50 ml round bottom flask that contained a magnetic stir bar. Approximately 10 ml of toluene was added to the flask. The mixture was sonicated for 1 min and then stirred while heated to reflux. The reflux mixture of GNRs and toluene was sonicated for 30 s. The reflux-sonication procedure was repeated 1–2 times to a total of 2–2.5 min of sonication time. Using a glass pipette, two drops of a GNR suspension were deposited on a substrate (either mica or Si/SiO 2 ) while still hot (>100 °C). Preparation of STM samples The suspension of GNR in toluene was prepared according to the above procedure. In order to prepare samples for the imaging of individual GNRs ( Figs 2c,d and 3g ) very dilute solutions of GNRs were used, which were sonicated with a higher intensity sonicator. An Au (111) single crystal sample was cleaned by repeated cycles of Ar + sputtering and annealing up to 700 °C. The substrate was imaged using an Omicron low-temperature STM (LT-STM) with electrochemically etched W tip to check for cleanliness, and the herringbone surface reconstruction was observed. The Au (111) single crystal was removed from vacuum and two drops of a GNR suspension were deposited on the substrate using a glass pipette. After ~5 min of drying in air, the sample was returned back to the UHV system. The prepared sample was annealed in 5 min increments at 40 °C to remove weakly bound surface adsorbates, for the total annealing time of 20 min. Preparation of samples for UV–vis-NIR spectroscopy Approximately 0.5 mg of a GNR powder was added to 5 ml of DMF. The GNR suspension was sonicated for 3 days before the measurements. Preparation of samples for photoluminescence spectroscopy Suspensions (0.167 mg ml −1 ) of monomer 3 , polymer 4 and GNRs 5 in dichloromethane were prepared. Polymer and GNR suspensions were sonicated for 15 min before the measurements. Preparation of samples for EDX and XPS Several droplets of a suspension of GNRs 5 in DCM was deposited on a gold foil and dried in air. Preparation of a sample for UPS/IPES measurements GNR powder was pressed in a pellet that was 0.75 cm in diameter and ~0.5 mm thick ( Supplementary Fig. 10 ). Raman spectrum simulation The Raman spectrum was simulated using the Quantum Espresso package [62] . Sample characterization 1 H and 13 C NMR was performed on Bruker 300 MHz, 400 MHz and 600 MHz NMR instruments. Magic angle spinning was performed at 600 MHz with the spinning speed of 8 kHz. AFM analysis was performed on a Digital Instruments Nanoscope IIIa Dimension 3100 system. AFM imaging was performed using Bruker RTESPA AFM probes (part # MPP-11120-10). Raman spectrum of GNRs was recorded on a Thermo Scientific DXR Raman Microscope with a 532 nm laser. UV–vis-NIR spectroscopy of performed on a Shimadzu UV-2401PC instrument. Photoluminescence spectra were obtained using a Shimadzu RF-5301PC instrument. Molecule 3 was characterized by MS using a Micromass GCT mass spectrometer with an electron impact (EI) direct probe that was heated up to 200 °C. Polymer 4 and GNRs 5 were analysed by matrix-assisted laser desorption/ionization (MALDI) MS on an Applied Biosystems Voyager DE-Pro instrument using a tetracyanoquinodimethane (TCNQ) matrix. EDX and SEM analysis was performed on a FEI Nova Nanosem 450 scanning electron microscope equipped with an Oxford Instruments EDX system. XPS was performed on a PHI Quantera SXM scanning X-ray microprobe. An Omicron LT-STM with an electrochemically etched W tip, kept at a base pressure of <10 −10 Torr, was used for the STM imaging. UPS/IPES measurements were performed using the home-build set-up described elsewhere [63] . The GNR pellet was placed on a Au (111) surface that was also used for the spectrometer calibration. The spectrometer was calibrated off the gold surface states, as is the position of the Fermi level in both photoemission and inverse photoemission; Supplementary Fig. 11 shows a UPS/IPES spectrum of Au (111). The energy dispersion was checked using shallow core levels or lanthanide compounds. The spectrometer resolution was determined off a 100 μm W or Ta wire. Since the photoelectron escape depth is <10 Å, and the probing inverse depth is <3 Å, while the GNR sample thickness was ~0.5 mm, we could not possibly observe any gold substrate features in the UPS/IPES spectra of GNRs. Therefore, there was no need for gold substrate background subtraction. How to cite this article: Vo, T. H. et al. Large-scale solution synthesis of narrow graphene nanoribbons. Nat. Commun. 5:3189 doi: 10.1038/ncomms4189 (2014).